Reversibility of anodic lithium in rechargeable lithium–oxygen batteries Non-aqueous lithium–air batteries represent the next-generation energy storage devices with very high theoretical capacity. The benefit of lithium–air batteries is based on the assumption that the anodic lithium is completely reversible during the discharge–charge process. Here we report our investigation on the reversibility of the anodic lithium inside of an operating lithium–air battery using spatially and temporally resolved synchrotron X-ray diffraction and three-dimensional micro-tomography technique. A combined electrochemical process is found, consisting of a partial recovery of lithium metal during the charging cycle and a constant accumulation of lithium hydroxide under both charging and discharging conditions. A lithium hydroxide layer forms on the anode separating the lithium metal from the separator. However, numerous microscopic ‘tunnels’ are also found within the hydroxide layer that provide a pathway to connect the metallic lithium with the electrolyte, enabling sustained ion-transport and battery operation until the total consumption of lithium. Rechargeable Li–O 2 batteries have attracted a great deal of attention recently as potential replacements for Li–ion batteries due to a higher theoretical capacity [1] , [2] , [3] , [4] , [5] , [6] , [7] , [8] , [9] , [10] , [11] , [12] , [13] , [14] . The advantage of Li–air cells over existing battery technologies lies in the very high-energy density of metallic Li (3,860 mAh g −1 ) through its electrochemical reaction with ambient oxygen. The basic assumption for the rechargeable Li–air battery hinges on that anodic lithium is completely reversible during the discharge–charge cycle. However, little is known experimentally on such reversibility at present. Although cell failure due to Li dendrite formation has been extensively studied for Li–ion battery application [15] , it is not clear if such a mechanism is applicable to the Li–O 2 batteries because of the differences in the cell construction, materials and operating environments. At present, the studies on the cyclability and stability of Li–O 2 batteries have been primarily focused on the cathode catalysts [16] , [17] , [18] , [19] , [20] , [21] , [22] , [23] , [24] , [25] , [26] , [27] , [28] , [29] , electrolytes [30] , [31] , [32] , [33] , [34] , [35] , [36] , [37] , [38] , [39] , [40] , [41] , [42] , [43] , [44] , binder [45] and so on. For example, the electrolyte decomposition was found during the cycling of Li–O 2 batteries, which led to the formation of by-products such as H 2 O, CO 2 , insoluble Li salts, and the eventual degradation of the cathode and the separator [33] , [34] , [35] , [36] , [46] , [47] , [48] , [49] , [50] , [51] . Research on anode stability is challenging due to the high reactivity of metallic Li. Any unintended exposure to the ambient environment during a postmortem analysis will alter the chemical state of the anode and the interpretation of the outcome. Furthermore, the result is most meaningful if the anodic behaviour is investigated in situ under the actual electrochemical conditions. We report herein an operando , spatially resolved phase and structural investigation on the lithium anode in an operating Li–O 2 cell using a micro-focused synchrotron X-ray diffraction (μ-XRD) technique. The changes in anode composition at different cycling stages and at various anode depths under multiple discharging-charging cycling are revealed for the first time. We find compound electrochemical processes involving partial recovery of metallic lithium during charging and continuous formation of lithium hydroxide (LiOH) during both charging and discharging steps. High-resolution, phase-contrast X-ray tomography is also employed to generate the three-dimensional (3D) morphologic image of the anode after multi-cycles in an attempt to understand its relevance to Li + transport in the anode. A large number of voids and holes are found in the LiOH layer, serving as lithium ion conducting channels to protract the battery cycling and lithium metal consumption. Lifespan of metallic Li anode in Li–O 2 cells Our study began with a multiple discharge–charge cycling test of a new Li–O 2 cell prepared with a carbon-black cathode, a lithium metal anode and a separator saturated with a LiCF 3 SO 3 /tetraethylene glycol dimethyl ether (TEGDME) electrolyte, which was extensively purified with H 2 O less than 8 p.p.m. The cell components were pre-baked at 50 °C before being assembled in the glove-box. 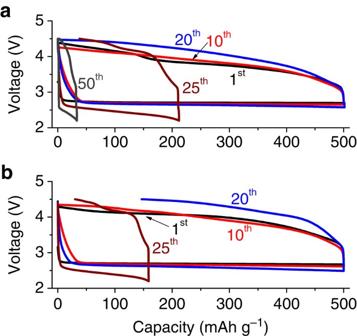Figure 1: Discharge–charge voltage profiles of Li–O2cells. (a) a new cell, (b) a ‘rebuilt’ cell using new cathode/separator but with used Li anode taken from the cell in (a) at the end of the cycling. Cycle numbers are marked by charging voltage curves. Figure 1a shows the cell’s voltage profiles of several representative cycles. During the first 10 cycles, the voltage profiles were stable. After the 20th cycle, the charging overpotential started to increase and the cell degradation accelerated. At the 50th cycle, the cell maintained less than 10% of initial capacity and was considered ‘failed’. The cell was subsequently dissected and was found still saturated with the liquid electrolyte, thus suggesting that electrolyte exhaustion was not the cause of the cell failure. The anode, on the other hand, was covered with a dark layer at its interface with the separator, whereas shiny metallic Li was still found on the current collector side (see Supplementary Fig. S1 ). Another cell was then rebuilt by incorporating this used Li anode covered by its black overlayer but with a new cathode/separator and fresh electrolyte. The rebuilt cell demonstrated nearly identical voltage profiles as the new one, as shown in Fig. 1b , suggesting the anode was still functioning and the loss of cyclability in Fig. 1a was primarily the result of the cathode deactivation. The rebuilt cell once again became deactivated after another round of multi-cycling and was disassembled for a second time. The anode showed a similar appearance to that observed at the end of first cycling test, except the dark layer became thicker and metallic layer appeared thinner. The above procedure was repeated several more times until the anode could no longer support regular cycling. At this point, the metallic shine of the anode completely disappeared. The total discharge capacity (105 C) summed from all the cycling experiments was found to be less than the theoretical capacity (167 C) of the Li foil (diameter 12 mm; thickness 0.20 mm). Figure 1: Discharge–charge voltage profiles of Li–O 2 cells. ( a ) a new cell, ( b ) a ‘rebuilt’ cell using new cathode/separator but with used Li anode taken from the cell in ( a ) at the end of the cycling. Cycle numbers are marked by charging voltage curves. Full size image Operando μ-XRD study of Li reversibility The above experiment clearly indicated that anodic lithium underwent an irreversible phase transformation during the cycling, although such a change did not interrupt the anode function significantly until the conversion was completed. To better understand the process and product of such conversion, a spatially resolved, operando μ-XRD experiment incorporating an operational Li–O 2 cell was designed. A schematic drawing of the experimental set-up, including the cell design, is shown in Fig. 2 . The cell was built using the same design and materials as the battery constructed for the discharge–charge cycling test, except with a smaller diameter (4.5 mm). During the experiment, discharge–charge cycling was carried out on the operando cell while X-ray diffraction patterns were collected layer-by-layer from the cathode to the anode with a spatial resolution of 20 μm. A control experiment on possible X-ray induced chemical change was also performed. All experimental details are presented in the Methods Section. 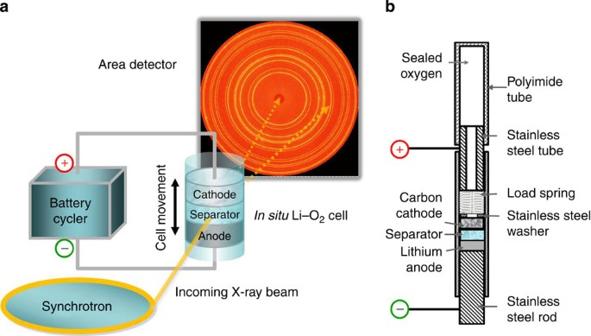Figure 2: The experimental set-up. (a)Operandoμ-XRD study of a Li–O2cell under cycling condition. (b) Cell schematic design. Figure 2: The experimental set-up. ( a ) Operando μ-XRD study of a Li–O 2 cell under cycling condition. ( b ) Cell schematic design. 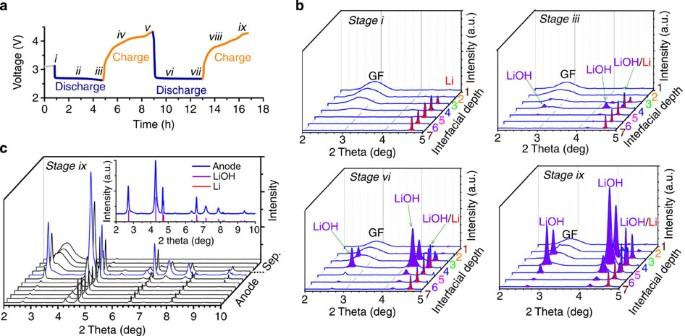Figure 3: The change in anodic lithium during discharge–charge cycling. (a) Discharge–charge voltage profile of theoperandoLi–O2cell as a function of cycling time. The stages at which XRD data sets were collected are marked asi, ii, iii… on the curve. (b) Four representative XRD sets taken at the cycling stagei, iii, vi, andix; each set consisted of seven selected XRD patterns collected at various anode–separator interfacial depths (marked as 1, 2, … 7 of different colours on the right of each set). (c) An expanded XRD data set at stageixcovering the whole anode through adjacent separator region. The inset is a representative XRD pattern taken from the position marked by a blue line that includes references of Li and LiOH. Full size image Figure 3a shows the voltage profile of the Li–O 2 cell operated at the synchrotron beamline. The battery first rested for 40 min at the open circuit potential followed by two discharge–charge cycles. During battery cycling, a total of nine sets of μ-XRD diffraction scans were taken at different discharging and charging stages with each set consisting of 30 XRD diffraction patterns collected at fixed intervals spanning the entire cell. The starting points for each data set, collected under different discharge/charge stages, are marked as i , ii , iii... on the cycling voltage profiles in Figure 3a . The acquisition time for each set took about 5 min. Fig. 3b shows four representative sets of XRD diffraction patterns (2°<2 θ <5°) at the cycling stage i (open circuit), iii (end of first discharge), vi (during second discharge) and ix (end of second charge). Only 7 of the full 30 scans are plotted to exemplify the change occurring at the interfacial region between the anode and the separator. The positions labelled as interfacial depth 3 and 4 represent the contact boundary between the anode and the separator, where both narrow metallic lithium peaks and broad glass fibre (GF) of the separator peaks are observed. (In the layered cell construction, we estimated the flatness of the Li-separator contact to be in the range of 20–30 μm over the diameter of 4.6 mm). Before commencing with the cycling, the lithium anode was in the metallic state, as is shown by the diffraction patterns of stage i in Fig. 3b , where the peaks in scan depth 3 to 7 (anode region) consisted of predominately Li metal diffraction peaks. As soon as the cycling started, the diffraction patterns changed. New features ascribed to LiOH started to emerge in the data sets of stage iii to ix, as the cycling progressed. An expanded set of XRD patterns (12 scans) acquired at the stage ix is also shown in Fig. 3c to provide a more complete view of the material composition at different anode depths. The inset in Fig. 3c shows a representative XRD spectrum taken from the anode and separator interfacial region with individual peak assignments. LiOH and metallic Li were the only two major phases identified in the XRD patterns. The presence of strong LiOH peaks near the separator interface indicates a significant conversion of Li-metal to LiOH. On the other hand, the metallic lithium remained the dominant crystalline phase deep inside of the anode on the current collector side. This observation suggests that the black layer previously observed was due to the presence of LiOH. Figure 3c also shows the weak but visible features of LiOH extended through the depth of the anode, which is attributed to the LiOH formed on the perimeter of the Li foil, as further witnessed by the black ring in Supplementary Fig. S1b . Figure 3: The change in anodic lithium during discharge–charge cycling. ( a ) Discharge–charge voltage profile of the operando Li–O 2 cell as a function of cycling time. The stages at which XRD data sets were collected are marked as i, ii, iii … on the curve. ( b ) Four representative XRD sets taken at the cycling stage i, iii, vi , and ix ; each set consisted of seven selected XRD patterns collected at various anode–separator interfacial depths (marked as 1, 2, … 7 of different colours on the right of each set). ( c ) An expanded XRD data set at stage ix covering the whole anode through adjacent separator region. The inset is a representative XRD pattern taken from the position marked by a blue line that includes references of Li and LiOH. Full size image The gradual conversion of metallic lithium to LiOH increased both the quantity and thickness of LiOH layer and reduced the amount of Li. The conversion continued as the discharge–charge cycling proceeded, as is shown by the LiOH intensity-thickness growths and reduction of Li in stage i through iX of Fig. 3b . 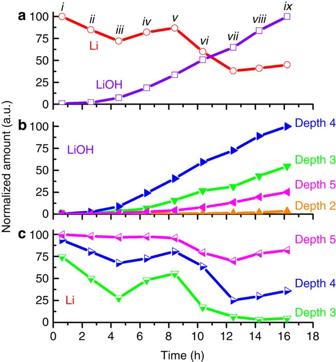Figure 4: Quantitative analysis of anode composition changes. (a) The overall change in the amount of LiOH and Li metal contents at the anode–separator interfacial region as a function of cycling time, individually normalized to the highest points of the respective components. The data collection positions (i, ii, iii … ix) during cycling were the same as those marked inFig. 3a. (b) Changes in the amount of LiOH at different interfacial depths (as marked by the scan number inFig. 3b) as a function of cycling time. The amounts at all depths are normalized to the highest intensity (depth 4 at 16th hour). (c) Changes in the amount of Li at different interfacial depths as a function of cycling time. The amounts at all depths are normalized to the highest intensity (depth 5 at beginning of cycling). Figure 4a shows the quantitative analysis of the LiOH and Li amounts as a function of cycling time, which was obtained by integrating the intensities of the changing Li and LiOH peaks at the interfacial region. First of all, we observed that after the depletion during the discharge (stage i through iii and v through vii ), the amount of metallic lithium was only partially recovered during the charging steps (stage iii through v and vii through ix ). In fact, only half of the lithium in the affected sample depth remained to be metallic after two cycles. The LiOH, on the other hand, increased monotonically in quantity and thickness during both discharge and charge steps. Figure 4b shows the integrated peak intensities of LiOH at interfacial depths 2 through 5 as a function of cycling time. Not only did the boundary-layer hydroxide concentration (depths 3 and 4) increase nearly linear with the cycling time, but also an appreciable amount of LiOH formed below (depth 5) and above (depth 2) the original lithium surface after the 8th and 14th hours, respectively. This growth indicates a continuous expansion of the hydroxide layer, both inward and outward, at the anode/separator interface. Using the Scherrer equation, the primary crystallite size of LiOH was found to remain nearly constant at 11 nm at different stages of the cycling depth. This observation suggests that LiOH, once formed, will not be dissolved or redeposited in subsequent charge or discharge reactions. We also analysed the change in Li-metal peak intensity at interfacial depths from 3 to 5, shown in Fig. 4c . All three layers showed a cyclic change in Li intensity with a gradual loss as the discharge–charge progressed. Due to its proximity to the electrolyte, the top layer lithium (depth 3) was affected the most and close to being depleted at the end of the second cycle. On the other hand, the loss and recovery of Li at depth 5 became only significant during the second cycle. The redeposited lithium during the charging step was most probably in the form of metal clusters with a broader diffraction bandwidth than the foil used as the fresh anode. As we will show in the following tomography study, however, the anodic Li surface was ‘pitted’ and no longer remained smooth once the cycling started, presumably as a result of different dissolution and deposition rates at different parts of the lithium surface during discharge–charge reactions. Under the circumstance, it was difficult to separate the peak width contributions by Li cluster or foil. Figure 4: Quantitative analysis of anode composition changes. ( a ) The overall change in the amount of LiOH and Li metal contents at the anode–separator interfacial region as a function of cycling time, individually normalized to the highest points of the respective components. The data collection positions ( i, ii, iii … ix ) during cycling were the same as those marked in Fig. 3a . ( b ) Changes in the amount of LiOH at different interfacial depths (as marked by the scan number in Fig. 3b ) as a function of cycling time. The amounts at all depths are normalized to the highest intensity (depth 4 at 16th hour). ( c ) Changes in the amount of Li at different interfacial depths as a function of cycling time. The amounts at all depths are normalized to the highest intensity (depth 5 at beginning of cycling). Full size image A longer cycling experiment (14 cycles) was also performed under the same conditions. As expected, the LiOH layer grew substantially thicker (see Supplementary Fig. S2 ). An ex situ μ-XRD study was also carried out for a failed, regular Li–O 2 cell, but only after the cell was ‘rebuilt’ and cycled a number of times using the same anode, as described for the process used in Fig. 1 . The metallic lithium at the anode was found to be completely converted to LiOH (see Supplementary Fig. S3 ). Last, we should point out that spatially resolved μ-XRD enabled the investigation of the individual sections of the battery without the interference by the other regions. In this case, for example, we found that LiOH existed only in the anode region under both in situ and ex situ experimental conditions. X-ray micro-tomographic study on anode morphology LiOH is neither an ion nor an electron conductor. Once it was formed on the metallic Li surface, how could the lithium metal continuously supply Li + to sustain the discharge–charge cycling? To address this question, we reconstructed a 3D microscopic image of a Li–O 2 cell using a non-destructive, synchrotron X-ray, phase-contrast micro-tomographic method. This method affords the morphological images at any given cross-section, thereby providing comprehensive, 3D structural information of the anode. The cell studied had been subjected to 14 cycles and was continuously operable, although a thick layer of LiOH (~140 μm) was observed on top of the anode, as was demonstrated by μ-XRD in Supplementary Figure S2 . 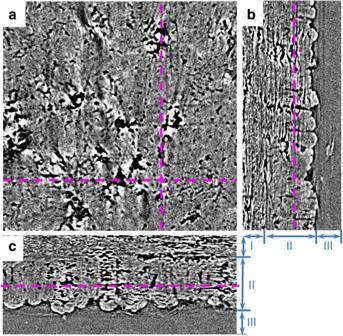Figure 5: X-ray tomography images of the used anode. (a) Planar cross-section of LiOH layer on the anode. (b,c) Vertical cross-sections through the anode, including a small portion of the separator. I: separator, II: LiOH layer and III: Li metal. The dimension of (a) is 823 μm × 806 μm. Images (b) and (c) have the same scale. Figure 5 shows three representative cross-sectional tomographic images taken from the anode. Figure 5a represents a planar top-view of the anode inside of the LiOH layer at the depth marked by the dashed lines in Fig. 5b,c , whereas Fig. 5b,c represents the side-views of the anode at the points marked by two dashed lines in Fig. 5a , respectively. Fig. 5b,c shows a thick coating of the LiOH on top of the Li metal. However, a significant number of holes and cracks are found in the LiOH layer, represented by the dark spots and shapes in Fig. 5a . These holes and cracks extend through the LiOH layer and are interconnected with each other throughout the LiOH layer, as shown in Fig. 5b,c . Figure 5: X-ray tomography images of the used anode. ( a ) Planar cross-section of LiOH layer on the anode. ( b , c ) Vertical cross-sections through the anode, including a small portion of the separator. I: separator, II: LiOH layer and III: Li metal. The dimension of ( a ) is 823 μm × 806 μm. Images ( b ) and ( c ) have the same scale. Full size image Complete anode morphology can be viewed in a video clip ( Supplementary Movie 1 ). The video starts at the separator region with the images of GFs. It then progresses into the LiOH layer where holes and cracks are visible. One can actually follow the holes and tunnels as the image frames move deeper into the anode layer until reaching the un-reacted lithium metal region. Selected frames of the video clip are also shown in Fig. 6 . On the top frame, the GF of the separator can be clearly seen at the separator–anode interface. The LiOH layer immediately underneath the separator shows large cracks and holes which are broken-out to smaller ones as the layers move deeper. Eventually, the porous hydroxide layer transitions to metallic Li with a smooth texture. The porous morphology with interconnected tunnels renders the liquid electrolyte continuously permeable through the LiOH layer to the lithium metal and maintained Li + transport. Therefore, the unused metallic Li can continue to supply Li + until it is totally consumed. We should point out that Figs 5 and 6 and Supplementary Movie 1 all show a well-defined boundary between LiOH and Li. No lithium dendrite formation is found, presumably due to inhibition by the hydroxide coating. 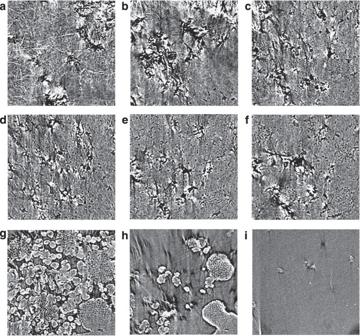Figure 6: Selected X-ray tomography images of anode. (a,b) the separator and anode interface; (c–f) LiOH layers; (g,h) breakout of LiOH at lithium metal interface; and (i) lithium metal layer. The depth separation between each frame is 20 μm. The dimension of each individual image is 800 μm × 790 μm. Figure 6: Selected X-ray tomography images of anode. ( a , b ) the separator and anode interface; ( c – f ) LiOH layers; ( g , h ) breakout of LiOH at lithium metal interface; and ( i ) lithium metal layer. The depth separation between each frame is 20 μm. The dimension of each individual image is 800 μm × 790 μm. Full size image Our investigation reveals limited anode reversibility in the Li–O 2 cell and a constant conversion of metallic Li to LiOH during both discharging and charging stages. In our ‘rebuilt’ cell study, all the anodic lithium metal was found to be consumed, but the total discharge capacity was less than the theoretical value of the metallic Li as a primary cell. Such discrepancy suggests the presence of non-electrochemical side reactions converting Li to LiOH, rendering it unavailable for discharge reaction. The most probable possibility, in our opinion, is through the reaction of lithium with water produced from the electrolyte decomposition. H 2 O would be produced as soon as the discharge–charge cycle started since it is a known by-product of decomposed ether-based electrolyte on cathodes [35] . Water is readily miscible with ether and can diffuse to the anode via the electrolyte to react with Li. As water is produced in both charge and discharge cycles, its reaction with lithium should be continuous and independent of the cycling stage, as we observed in this experiment. Although the cathodic cyclability has been extensively investigated for Li–O 2 batteries containing different electrolytes, our study brings forth a fundamental concern on the anode rechargeability when the electrolyte stability is an issue. Another important observation by our spatially resolved μ-XRD study is that LiOH distributes exclusively in the anode region. This is particularly interesting as water is presumably formed through electrolyte decomposition at the cathode, where lithium peroxide is readily available as the discharging product. Clearly, more experimental and theoretical investigations are needed to understand the interdependence between the electrochemical and chemical reactions inside the Li–air battery. In summary, the conversion of metallic lithium to LiOH on the anode is observed using micro-focused, synchrotron X-ray diffraction and phase-contrast X-ray tomography methods during discharge–charge cycling of Li–O 2 cells. The Li metal in the anode is found to have very limited reversibility, whereas the thickness of LiOH layer increases steadily as the cycling progressed, possibly resulting from the reaction of Li with H 2 O formed through the electrolyte decomposition. Li + transport is maintained through porous channels in the LiOH layer until the metallic lithium is completely consumed. This study demonstrate a general degradation process at the anodes associated with the current non-aqueous Li–O 2 batteries. It should further motivate the development of a stable, decomposition-free electrolyte that could mitigate the issue at both electrodes. Li–O 2 battery assembly and test The cathode was prepared by mixing carbon black (Black Pearl 2000, Cabot) and polyvinylidene fluoride, used as a binder, with an 80/20 weight ratio. The cathode slurry was brushed onto circular carbon papers (diameter=11 mm) and dried at 80 °C overnight in a vacuum oven before being assembled into the batteries. The carbon loadings were 0.5~1 mg cm −2 . Li–O 2 batteries were assembled inside of an Ar-filled glove-box using a Swagelok-type cell construction. A circular Li foil with a diameter of 12 mm was used as the anode. Between the anode and the cathode was a separator prepared by glass microfibre filter (Whatman, GF/F, 150) soaked with 150 μl of electrolyte: 1 M LiCF 3 SO 3 /TEGDME. TEGDME was procured from Aldrich and purified extensively by distillation and molecular sieve before use. The water content in the purified electrolyte was less than 8 p.p.m. Each Li–O 2 battery was encapsulated in a tubular glass cell. All the cell components were kept in drying oven at 50 °C before being transferred to Ar-filled glove-box for the cell assembly. The cell was first purged with ultrahigh purity oxygen for 30 min before being sealed at 1 atm. The discharge–charge cycling of the cells was controlled by a MACCOR system under a current density of 0.05 mA cm −2 . Discharge–charge duration was controlled at 5 h, respectively. For the in situ cells used in the μ-XRD and X-ray tomographic experiments, the cell diameter was reduced to 4.5 mm. The current was 0.02 mA and the duration was 4 h for both discharge and charge cycle during the operando study. μ-XRD and micro-tomography experiments The μ-XRD and micro-tomography experiments were conducted using a high-energy (60.5 keV) X-ray beam at the 1-ID-C beamline of the Advanced Photon Source, Argonne National Laboratory [52] , [53] . Two-dimensional diffraction patterns were collected using an amorphous-Si area detector. Tomographic data were collected using a high-resolution area detector. For μ-XRD experiment, the 20-μm vertical beam size was achieved by focusing with Si saw tooth refractive lenses using an experimental set-up previously reported [54] . Inside of an Ar-filled glove-box, a cylindrically-shaped cell containing a sandwich of cathode (diameter 4.5 mm), separator (diameter 4.5 mm) and anode (diameter 4.0 mm) was assembled inside of a polyimide tube (ID: 4.5 mm). All the cell components except lithium foil were first baked at 50 °C for 24 h before being transferred to the glove-box for assembly. On the cathode side, the cell was connected to a tube filled with oxygen of ultrahigh purity. Each electrode was connected to the respective poles of a cycler, which controlled the discharge–charge cycling experiment. Although the diameter of the cell was thinner than our regular cells for high angular resolution of the diffraction peaks, the voltage profiles are essentially the same between the two. The Li–O 2 battery was mounted on a high-precision translational stage at the synchrotron beamline, and the cylindrical axis was normal to the micro-focused X-ray beam. The layer-by-layer X-ray scattering from different positions between the cell’s electrodes was collected by moving the battery vertically at 20 μm per step. The X-ray exposure at each scan position was 10 s. The total X-ray exposure time for each set, which covered from cathode, separator and anode, was about 5 min. The X-ray scattering patterns were systematically acquired by the area detector that was calibrated using a CeO 2 standard. The patterns collected for different cell positions were then integrated after subtraction of dark current and background noise. For operando Li–O 2 battery experiments, there is a concern that the electrolyte, upon absorption of X-ray photons, may undergo a photon-induced decomposition reaction. Such a reaction, if present, would affect the result from the electrochemical reaction. A control experiment was carried out in which a Li–O 2 cell was subjected to the identical X-ray exposure and scan pattern as that described for the experiment in Fig. 3 . The only difference was that the cell was kept at open circuit voltage so that no electrochemical reaction occurred. No change on the anode was observed. This control study indicates that the result of this operando measurement was not altered by X-ray radiation. This is mainly due to relatively low absorption by the battery-electrolyte materials of the very high-energy X-rays used in the current study. At 60.5 keV, the absorption of X-ray by the major elements in the electrolyte such as C or O is about two and four order of magnitudes lower than that at 10 and 1 keV, respectively [55] , which explains why no X-ray-induced decomposition was observed. (see Supplementary Fig. S4 ) In parallel beam micro-tomography measurements, the sample was centred to the rotation axis and rotated through 180°, acquiring projection images at 0.2° intervals. To cover the entire cell, we used the so called wide field-of-view tomography technique by dividing up the sample width by several field-of-views. In this experiment we used a 60.5 keV X-ray beam that had sufficient penetration through the 4.5 mm thick battery cell. In order to have full coverage over the entire cell, we applied three 1.9 mm × 1 mm irradiated areas with 200 μm overlaps which were necessary for the correct stitching of the adjacent projections. The thickness of the LuAG:Ce single-crystal scintillator was 25 μm, which produced the visible photons for the × 7.5 objective and the 2048 × 2048 pixel charge-coupled device camera. According to the thin scintillator, the overall spatial resolution of this tomography set-up was about 2–3 μm with 1 μm pixel size. The sample-detector distance was 470 mm in order to obtain both phase contrast and absorption contrast. The phase-contrast imaging enabled us to make the interfaces of the different components in the cell with similar X-ray absorption clearly distinguishable. How to cite this article: Shui, J.-L. et al . Reversibility of anodic lithium in rechargeable lithium–oxygen batteries. Nat. Commun. 4:2255 doi: 10.1038/ncomms3255 (2013).